Improved nucleosome-positioning algorithm iNPS for accurate nucleosome positioning from sequencing data Accurate determination of genome-wide nucleosome positioning can provide important insights into global gene regulation. Here, we describe the development of an improved nucleosome-positioning algorithm—iNPS—which achieves significantly better performance than the widely used NPS package. By determining nucleosome boundaries more precisely and merging or separating shoulder peaks based on local MNase-seq signals, iNPS can unambiguously detect 60% more nucleosomes. The detected nucleosomes display better nucleosome ‘widths’ and neighbouring centre–centre distance distributions, giving rise to sharper patterns and better phasing of average nucleosome profiles and higher consistency between independent data subsets. In addition to its unique advantage in classifying nucleosomes by shape to reveal their different biological properties, iNPS also achieves higher significance and lower false positive rates than previously published methods. The application of iNPS to T-cell activation data demonstrates a greater ability to facilitate detection of nucleosome repositioning, uncovering additional biological features underlying the activation process. The technology of micrococcal nuclease (MNase) digestion combined with high-throughput sequencing (MNase-seq) is a powerful method to map the genome-wide distribution of nucleosome occupancy [1] , [2] , [3] . Although it has a high demand on sequencing depth, with the promise of probing whole genome-wide chromatin remodelling events incurred by all transcription factor binding and chromatin modifications at once and the rapidly decreasing sequencing cost, its popularity has continued to increase over the years. However, the analysis of nucleosome positions is still at its infancy. Nucleosome positioning relies on nucleosome signal coverage, or the frequency distribution formed by MNase digested DNA fragments in a cell population. A genome location where there is nucleosome occupancy in a number of cells would have high sequencing read coverage. Thus, the essential principle for nucleosome position detection is to find the locations where the MNase-seq coverage is enriched. An effective and efficient strategy is to generate a nucleosome sequencing profile that is able to intuitively depict the nucleosome distribution in a wave-form, based on which a peak-calling procedure is then used to find the peaks on the wave-form profile. Zhang et al . [4] have developed an algorithm for nucleosome detection called nucleosome positioning from sequencing (NPS). 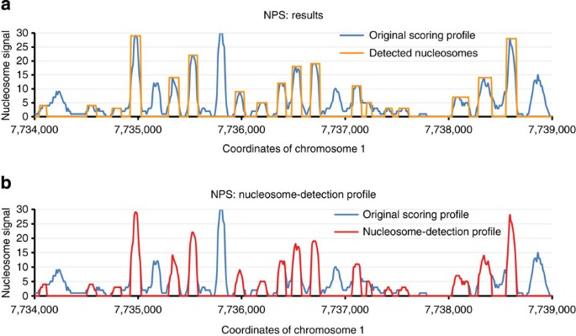Figure 1: Nucleosomes detection results by the NPS algorithm. (a,b) The nucleosome detection results of the NPS algorithm on the 7,734,000–7,739,000 bp region of chromosome 1 (hg18) in resting human CD4+ T cells. (a) The detected nucleosomes (orange line). (b) The nucleosome-detection profile (red line): wave-form signal within the detected nucleosomes. In practice, however, the accuracy of the NPS algorithm [4] needs much improvement: even if the thresholds for all the filtering steps in the programme are lowered or eliminated ( Supplementary Table 1 ), many visually obvious nucleosomes still could not be detected. To solve this problem, we first identified the technical problems in NPS contributing to the missing or mis-detected nucleosomes; then, we developed a new package ‘improved NPS’ (iNPS) by combining the theoretical core algorithm of NPS [4] with new algorithms to address these technical problems. iNPS exhibits a remarkably improved performance over the original NPS, detecting nucleosomes with higher quality, a lower false positive rate and stronger association with relevant biological events. We also find that NPS’ deficiency can be largely traced to a hard-coded parameter ( Supplementary Fig. 1a,b ); yet, the performance of iNPS is still significantly better than the ‘customized NPS’ that has the hard-coding problem fixed ( Supplementary Fig. 1c ). In addition to the NPS comparison (both default and customized NPS), we further demonstrated an overall advantage of iNPS over other recent algorithms used for nucleosome detection. In particular, iNPS has a unique advantage of detecting different types of nucleosomes that are associated with different biological properties based on detected nucleosome shapes. The significant increase in accuracy of the iNPS algorithm tackled the previously thought major limitations of the MNase-seq technology, namely its low resolution and low consistency in nucleosome boundary determination [5] . We now demonstrate that the limitations do not lie so much in the technology per se , but rather lie in the accuracy of the computational analysis method. The iNPS software package is freely downloadable at http://www.picb.ac.cn/hanlab/iNPS.html . Improved nucleosome positioning from MNase-seq data The original NPS algorithm [4] mainly contains the following four steps: (1) nucleosome scoring for generating a continuous wave-form signal for a distribution profile of genome-wide nucleosome positioning, (2) wavelet denoising for the preliminary mild smoothing of the signal waves, (3) Laplacian of Gaussian convolution (LoG) for further smoothing the wave profile and meanwhile detecting inflection points on the profile as the borders of nucleosome peaks and (4) peak filtering based on the cutoff of peak shape and the P -value of Poisson approximation. In NPS, the original nucleosome profile was generated by extending each MNase-seq tag from the 5′ end by 150 bp towards the 3′ position and taking the middle 75 bp as the enriched nucleosome signal, thus the nucleosomes were represented by the peaks on the wave-like original profile. Borders of the nucleosome peaks, represented by paired inflection points on the smoothed profile, could be detected by LoG (Methods). However, the original NPS algorithm cannot precisely determine which pairs of inflection points should be selected as final nucleosomes; thus, as false positives, some mildly concave parts are determined as nucleosome positions while some obvious sharp peaks are missed ( Fig. 1a,b ). To solve this problem, our iNPS algorithm used a new method, the first derivative of Gaussian convolution, for detecting max/min-extremum points to identify each inflection point pair as ‘main’ nucleosome peaks or ‘shoulders’ (Methods, Fig. 2a ). This new step is based on the observation that a sharp peak has a summit on the smoothed profile, while a mildly concave shoulder does not. Then, this step was followed by the next new step for determining whether a ‘shoulder’ candidate should be an independent nucleosome or merged into the neighbouring ‘main’ nucleosome candidate that has a dynamic shift. Here, the determination depends on the distance between the shoulder and the main peaks, their peak height ratio, and, particularly, the profile shape features between the nearest inflection point on the adjacent ‘main’ nucleosome peak and the ‘most-winding’ point (detected by the third derivative of Gaussian convolution) on the ‘shoulder’ (Methods, Fig. 2a , and see examples in Supplementary Fig. 2 ). Following these two new major improvements to assure the accuracy of detecting the ‘main’ nucleosome peaks, fine adjustments were made, including adjusting nucleosome border, merging ‘doublets’, and so on, to resolve minor peaks. On the basis of these improvements, we developed a high-accuracy nucleosome-positioning algorithm, the iNPS algorithm ( Fig. 2b and see an example of step-by-step optimization in Fig. 2c , and also see an example of the detection result by NPS in Fig. 2d for comparison). Figure 1: Nucleosomes detection results by the NPS algorithm. ( a,b ) The nucleosome detection results of the NPS algorithm on the 7,734,000–7,739,000 bp region of chromosome 1 (hg18) in resting human CD4+ T cells. ( a ) The detected nucleosomes (orange line). ( b ) The nucleosome-detection profile (red line): wave-form signal within the detected nucleosomes. 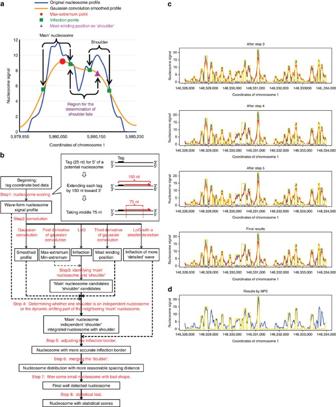Figure 2: The algorithmic procedure of iNPS. (a) An illustration of the relationship between a ‘main’ nucleosome and a ‘shoulder’ pattern. (b) Flow chart of the seven algorithmic steps in iNPS. (c) Step-by-step results of iNPS algorithm. Genomic region 148,328,000–148,334,000 bp in chromosome 1, hg18 of human resting CD4+ T cells is used here as an example. Five coloured profile lines are plotted in each panel–blue: original scoring profile, red: Gaussian convolution smoothed profile, green/purple: LoG convoluted profiles with normal/smaller standard deviations, orange: detected nucleosome peaks. Results after step 3: detection of candidate ‘main’ nucleosomes/‘shoulders’ (that is, the region of a pair of inflection points with/without max-extreme point between them). Results after step 4: ‘shoulders’ are determined as independent nucleosomes or dynamic shifting parts of the neighbouring main nucleosome peaks. Results after step 5: borders of some nucleosomes are adjusted using inflection points identified from the LoG convoluted profiles with a small standard deviation. Final results: ‘doublets’ patterns are merged and small nucleosome peaks with bad shapes are discarded. (d) The final nucleosome detection result by NPS on the same genomic region as inc. Full size image Figure 2: The algorithmic procedure of iNPS. ( a ) An illustration of the relationship between a ‘main’ nucleosome and a ‘shoulder’ pattern. ( b ) Flow chart of the seven algorithmic steps in iNPS. ( c ) Step-by-step results of iNPS algorithm. Genomic region 148,328,000–148,334,000 bp in chromosome 1, hg18 of human resting CD4+ T cells is used here as an example. Five coloured profile lines are plotted in each panel–blue: original scoring profile, red: Gaussian convolution smoothed profile, green/purple: LoG convoluted profiles with normal/smaller standard deviations, orange: detected nucleosome peaks. Results after step 3: detection of candidate ‘main’ nucleosomes/‘shoulders’ (that is, the region of a pair of inflection points with/without max-extreme point between them). Results after step 4: ‘shoulders’ are determined as independent nucleosomes or dynamic shifting parts of the neighbouring main nucleosome peaks. Results after step 5: borders of some nucleosomes are adjusted using inflection points identified from the LoG convoluted profiles with a small standard deviation. Final results: ‘doublets’ patterns are merged and small nucleosome peaks with bad shapes are discarded. ( d ) The final nucleosome detection result by NPS on the same genomic region as in c . Full size image As a result of introducing these aforementioned steps, the iNPS algorithm detected more nucleosomes than NPS, among which many obvious sharp peaks missed by NPS are retrieved (Compare Fig. 3a,b versus Fig. 1a,b ). The full list of genomic coordinates and shape features of the exemplary nucleosomes detected ( Fig. 3a,b ) are listed in Supplementary Table 2 . 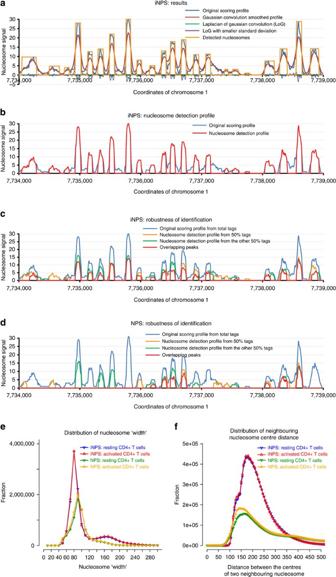Figure 3: Improved nucleosome detection results by iNPS. (a–d) Genomic region 7,734,000–7,739,000 bp (hg18) of chromosome 1 in human resting CD4+ T cells is shown as an example. (a) Nucleosome detection results by iNPS. (b) The nucleosome detection profile (wave-form signal within detected nucleosomes) by iNPS (red line). (c) Robustness of iNPS’s detection results. The SCC between nucleosome detection profiles derived from two sub-data sets (orange and green line) is 0.681. (d) Robustness of NPS’s detection results. The SCC between the nucleosome detection profiles derived from two sub-data sets (orange and green line) is 0.417. (e) Distribution of nucleosome ‘width’—the length between two inflection points of each detected nucleosome. (f) Distribution of the distance between the centre points of two neighbouring nucleosomes. Figure 3: Improved nucleosome detection results by iNPS. ( a – d ) Genomic region 7,734,000–7,739,000 bp (hg18) of chromosome 1 in human resting CD4+ T cells is shown as an example. ( a ) Nucleosome detection results by iNPS. ( b ) The nucleosome detection profile (wave-form signal within detected nucleosomes) by iNPS (red line). ( c ) Robustness of iNPS’s detection results. The SCC between nucleosome detection profiles derived from two sub-data sets (orange and green line) is 0.681. ( d ) Robustness of NPS’s detection results. The SCC between the nucleosome detection profiles derived from two sub-data sets (orange and green line) is 0.417. ( e ) Distribution of nucleosome ‘width’—the length between two inflection points of each detected nucleosome. ( f ) Distribution of the distance between the centre points of two neighbouring nucleosomes. Full size image The distribution of nucleosome ‘width’, as represented by the length between two inflection points of each detected nucleosome peak, is plotted in Fig. 3e . It is clear that for most nucleosomes, the ‘width’ is around 70–90 bp, which is consistent with the fact that the middle 75 bp of extended tags was taken to represent the enrichment signal of a nucleosome. The sharp peak of the nucleosome width distribution suggests that the majority of the detected nucleosomes are well-positioned and isolated single nucleosomes. Furthermore, the distances between the centres of two neighbouring nucleosomes are around 160–210 bp, peaking at 180 bp ( Fig. 3f ). This distance distribution is consistent with the fact that nucleosomes are wrapped by a stretch of 147 bp of DNA and separated by ~38 bp of linker DNA [6] . We then specifically assessed the influence on the distributions and average nucleosome profiles by different parts of the iNPS pipeline. By sequentially activating each algorithmic step (including substeps of Step 6: merging ‘doublets’ and Step 7: filtering) of iNPS, we observed an increasingly sharper distribution of nucleosome widths ( Supplementary Fig. 3a ), an increasingly better approximation of the neighbouring nucleosome centre distance to the theoretical value (147 bp nucleosome+38 bp linker) ( Supplementary Fig. 3b ) and increasingly sharper peaks/better phasing of the average nucleosome profiles ( Supplementary Fig. 3e ) from Step 3 to Step 7 on chromosome 1 of the resting CD4+ T cells. We also observed a mild decreasing of the number of output nucleosomes through these steps ( Supplementary Table 3 ). The analysis of the distribution of nucleosome ‘width’ and neighbouring nucleosome centre distance was also repeated on Chromosome 19 of activated CD4+ T cells. The results are qualitatively similar and shown in Supplementary Fig. 3c,d . In contrast, the original NPS algorithm results in a much more diffuse and flattened distribution of the nucleosome width (peaking around 70–110 bp) ( Fig. 3e ) and the neighbouring centre distance (around 130–180 bp, peaking at 150 bp) ( Fig. 3f ). Therefore, the comparison suggests that our iNPS algorithm is able to detect a larger number of well-fixed and well-isolated nucleosomes with a more precise centre distance between neighbouring nucleosomes. Moreover, the distributions generated by iNPS are more consistent between human resting and activated CD4+ T cells compared with those generated by NPS ( Fig. 3e,f ). Although the customized NPS shows better performance than the original default NPS ( Supplementary Fig. 4a,b versus Fig. 1a,b ), its performance is still not as good as iNPS, as shown by the distribution of nucleosome width, the distribution of neighbouring centre distance, and the consistency between resting and activated T cells ( Supplementary Fig. 4d,e ). Quality of genome-wide nucleosome detection For each detected nucleosome, iNPS scores the confidence level using Poisson test as applied by NPS [4] and some other peak-calling algorithms for ChIP-seq data, such as MACS [7] . Unlike NPS and MACS, iNPS not only identifies the tag enrichment within the peak region (see definition in Methods) for each detected nucleosome peak by using upper-tailed Poisson test, but it also identifies the tag depletion within the adjacent ‘valley’ regions (see definition in Methods) flanking the corresponding nucleosome peak by using lower-tailed Poisson test, resulting in two respective scores ‘−log10( P -value_of_peak)’ and ‘−log10( P -value_of_valley)’ (see ‘Step 8’ of ‘Algorithmic steps in iNPS’ in Methods for details). We compared the genome-wide quality of nucleosome output by iNPS/NPS by performing Poisson tests for all the detected nucleosomes and by sorting them in decreasing order of ‘−log10( P -value_of_peak)’ and ‘−log10( P -value_of_valley)’, respectively. Then, the average −log10( P -value) of nucleosomes (per 10,000-sized bins) are plotted for the top 5,000,000 predicted nucleosomes by iNPS or NPS on the whole genome of the resting and activated CD4+ T cells, respectively ( Fig. 4a,b ). It is clear that iNPS outperforms NPS. 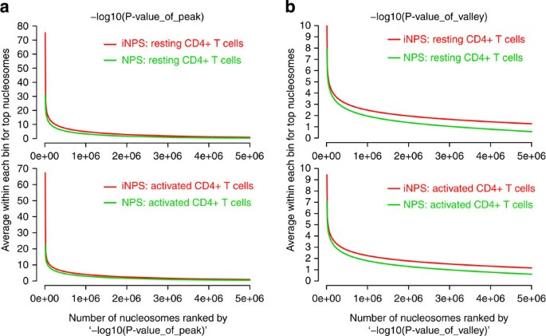Figure 4: Comparing the quality of nucleosomes detected by iNPS and NPS. (a,b) Significance of the peak/valley regions of the detected nucleosomes, quantified by ‘−log10(P-value_of_peak)’ (a) and ‘−log10(P-value_of_valley)’ (b). The genome-wide MNase-seq data of both resting and activated CD4+ T cells are used, and the −log(P-value) of the top 5,000,000 nucleosomes ranked by ‘−log10(P-value_of_peak)’ (a) and ‘−log10(P-value_of_valley)’ (b) are plotted with each bin showing the averaged value of 10,000 nucleosomes. Figure 4: Comparing the quality of nucleosomes detected by iNPS and NPS. ( a,b ) Significance of the peak/valley regions of the detected nucleosomes, quantified by ‘−log10( P -value_of_peak)’ ( a ) and ‘−log10( P -value_of_valley)’ ( b ). The genome-wide MNase-seq data of both resting and activated CD4+ T cells are used, and the −log( P -value) of the top 5,000,000 nucleosomes ranked by ‘−log10( P -value_of_peak)’ ( a ) and ‘−log10( P -value_of_valley)’ ( b ) are plotted with each bin showing the averaged value of 10,000 nucleosomes. Full size image In addition, we also evaluated the genome-wide detection quality of the customized NPS, which is better than the default NPS (the blue lines versus green lines in Supplementary Fig. 5 ), as expected. However, iNPS still yields overall higher −log( P -value) scores (the red lines versus blue lines in Supplementary Fig. 5 ) than customized NPS, demonstrating the best quality of the detected nucleosomes by iNPS. Robustness of genome-wide nucleosome detection To compare the robustness of the nucleosome detection by iNPS and NPS, we randomly and evenly divided the MNase-seq data [1] into two subsets (50% tags in each subset) and obtained two nucleosome detection results by running iNPS and NPS with the same parameter settings on the two data sets (Methods). Then, the robustness of the algorithms was quantified by Spearman’s rank correlation coefficient (SCC) between results on the two independent subsets of the data to measure their similarity (Methods). Using the DNA fragment of Figs 1 and 3 as an example, the SCC for iNPS-derived profiles (measuring the similarity of the orange and green lines in Fig. 3c ) is 0.681, while the SCC of NPS and customized NPS-derived profiles (measuring the similarity of the orange and green lines in Fig. 3d and Supplementary Fig. 4c ) is 0.417 (NPS) and 0.635 (customized NPS), respectively. At the whole-genome level, the differences in SCCs between detections on two halves of tags across each of the 24 human chromosomes (1–22, X and Y; Fig. 5a , Supplementary Fig. 6 and Supplementary Table 4 ) are highly significant (average±s.d. are 0.489±0.029, 0.339±0.039 and 0.444±0.042 for iNPS, NPS, and customized NPS, respectively, with one-tailed paired t -test P =3.37 × 10 −21 between iNPS and NPS, P =8.76 × 10 −9 between iNPS and customized NPS). 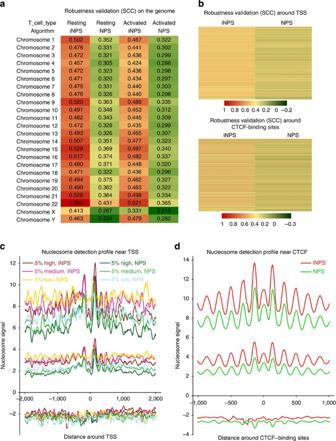Figure 5: Comparison of the robustness and average profiles of nucleosome detection by iNPS and NPS. (a) Heatmap of SCCs between the ‘nucleosome detection profiles’ derived from the two independent subsets containing 50% tags each. SCCs are calculated for the whole genome and for every chromosome (1–22, X and Y) in both resting and activated CD4+ T cells. (b) Similar toa, but the SCCs are computed over regions around TSS/CTCF-binding sites in human resting CD4+ cells. (c) The average nucleosome detection profiles with s.d. by NPS and iNPS. Three sets of genes are selected according to high, medium and low transcription levels. For each set, the average and s.d. of the signals at 10 bp resolution are plotted in warm/cold colours to represent the corresponding nucleosome detection results by iNPS/NPS. The lines in the middle: average profiles of detected nucleosomes; the lines in the upper and lower parts of the figures are the average±s.d. profiles for the iNPS/NPS results. (d) Average nucleosome profiles with s.d. at CTCF regions by iNPS/NPS. Figure 5: Comparison of the robustness and average profiles of nucleosome detection by iNPS and NPS. ( a ) Heatmap of SCCs between the ‘nucleosome detection profiles’ derived from the two independent subsets containing 50% tags each. SCCs are calculated for the whole genome and for every chromosome (1–22, X and Y) in both resting and activated CD4+ T cells. ( b ) Similar to a , but the SCCs are computed over regions around TSS/CTCF-binding sites in human resting CD4+ cells. ( c ) The average nucleosome detection profiles with s.d. by NPS and iNPS. Three sets of genes are selected according to high, medium and low transcription levels. For each set, the average and s.d. of the signals at 10 bp resolution are plotted in warm/cold colours to represent the corresponding nucleosome detection results by iNPS/NPS. The lines in the middle: average profiles of detected nucleosomes; the lines in the upper and lower parts of the figures are the average±s.d. profiles for the iNPS/NPS results. ( d ) Average nucleosome profiles with s.d. at CTCF regions by iNPS/NPS. Full size image To further compare the three algorithms using another independent dataset, we ran a similar analysis on the MNase-seq data for activated CD4+ T cells. The SCCs (average±s.d.) for iNPS, NPS and customized NPS are 0.454±0.036, 0.309±0.028 and 0.409±0.036, respectively (one-tailed paired t -test P =1.99 × 10 −24 between iNPS and NPS and P =2.07 × 10 −11 between iNPS and customized NPS, Fig. 5a , Supplementary Fig. 6 and Supplementary Table 4 ). As background controls, we calculated the SCCs expected from random simulations on chromosome 1 by randomly selecting ‘detected nucleosomes’ with the same number and total coverage length of the two real nucleosome detection ‘subresults’ given by iNPS. They have an average±s.d. of 0.113±0.00046 based on 100 times permutations, giving rise to an empirical P -value <0.01 for iNPS-derived SCCs. We also performed a genome-wide simulation across all the 24 chromosomes (1–22, X and Y), the results are similar to that of the 100 simulations on Chromosome 1 (average SCC±s.d.=0.105±0.015). In addition, since nucleosomes are well phased at TSS and CTCF-binding sites, we specifically tested the robustness of the two algorithms in the regions of TSS (−2,000 to +2,000 bp) and CTCF (−1,000 to +1,000 bp) in the resting CD4+ T cell. The results are similar to those obtained at the single chromosome level ( Fig. 5b ). Average profiles of detected nucleosomes We then examined the differences between the average nucleosome detection profiles obtained by retaining only the wave-signal within the nucleosome peaks detected by NPS and iNPS (See the red line in Fig. 1b versus Fig. 3b for an example). From the average profiles and the s.d. derived from the two algorithms surrounding TSSs (which are further classified according to high, medium and low gene transcription levels) and CTCF-binding sites ( Fig. 5c,d ; see also Supplementary Fig. 7 and Supplementary Fig. 8 for more examples), we can clearly observe the following key differences between the profiles generated by the two algorithms. (1) For iNPS, the average nucleosome distributions around TSSs at the three expression levels are clearly separated and consistent with the expression levels. Even at TSSs of lowly expressed genes, the nucleosome phasing can still be observed, whereas NPS gives no signal for TSSs of lowly expressed genes, and the differences between the profiles for medium and high levels are not as distinctive ( Fig. 5c ). (2) The nucleosome peaks detected by iNPS are sharper than those by NPS (See examples in Supplementary Fig. 7 ). (3) The s.d. profiles (s.d. of the signals at each 10 bp interval within the TSS±2 kb region) by iNPS also have larger fluctuations than NPS ( Fig. 5c ), indicating that iNPS is more sensitive in identifying the boundary of nucleosomes with different shapes. (4) Similar to these improvements at the TSSs, at CTCF-binding sites, both the average and s.d. profiles of nucleosomes detected by both algorithms support remarkable performance improvements of iNPS versus NPS ( Fig. 5d , and see examples in Supplementary Fig. 8 ). Differential nucleosome positioning As transcription factor binding and chromatin remodelling are associated with the change of nucleosome positions or occupancies [8] , [9] , we investigated the differentially positioned nucleosomes between resting and activated CD4+ T cells (see pipeline in Supplementary Fig. 9 ). The MNase-seq tags contributing to the iNPS-detected nucleosomes were selected and inputted into DANPOS [10] to obtain differentially positioned nucleosomes (Methods, see the example fragment in Fig. 6a ) for the analysis of biological significance (Methods). Among the Top 30 enriched pathways and transcription factor binding motifs ( Fig. 6b ), several are associated with the T-cell activation, such as ‘Sphingosine 1-phosphate (S1P) pathway’ [11] , [12] , ‘Integrin family cell surface interactions’ [13] , ‘LKB1 signalling events’ [14] , [15] , [16] , ‘Proteoglycan syndecan-mediated signalling events’ [17] , ‘TRAIL signalling pathway’ [18] , ‘VEGF and VEGFR signalling network’ [19] , ‘IL3-mediated signalling events’ [20] and motif (‘ TGGAAA ’) for NFAT transcription factor family (nuclear factor of activated T cells) binding. Moreover, the largest network component connecting these transcription factors is significantly larger than random expectation (Methods, Fig. 6c,d , size of 62 nodes versus an average of 21 nodes of 10,000 randomly constructed networks among the same number of proteins, empirical P -value <10 −4 ). Finally, co-citation analysis suggested that iNPS-derived transcription factors yields high average PubMed counts (6.542) with a significant P -value ( P <0.001), showing significant biological correlation with T-cell activation (Methods). 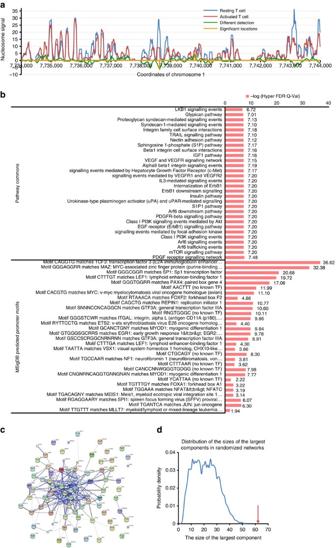Figure 6: Analysis of differential nucleosome positioning between the resting and activated CD4+ T cells revealed by iNPS. (a) An exemplary genomic region shows the differential nucleosome positioning based on iNPS’ results in the resting and activated T cells. (b) Top enriched pathways and ‘MSigDB Predicted Promoter Motifs’ associated with genomic regions showing differential nucleosome positioning between the resting and activated CD4+ T cells. (c) The network among transcription factors with at least one of the most enriched ‘MSigDB Predicted Promoter Motifs’ (hypergeometric test FDR <0.001 output by GREAT). (d) Distribution of the sizes of the largest components in randomized networks, with the size of the largest network component incmarked by the arrow. Figure 6: Analysis of differential nucleosome positioning between the resting and activated CD4+ T cells revealed by iNPS. ( a ) An exemplary genomic region shows the differential nucleosome positioning based on iNPS’ results in the resting and activated T cells. ( b ) Top enriched pathways and ‘MSigDB Predicted Promoter Motifs’ associated with genomic regions showing differential nucleosome positioning between the resting and activated CD4+ T cells. ( c ) The network among transcription factors with at least one of the most enriched ‘MSigDB Predicted Promoter Motifs’ (hypergeometric test FDR <0.001 output by GREAT). ( d ) Distribution of the sizes of the largest components in randomized networks, with the size of the largest network component in c marked by the arrow. Full size image The same analysis was also performed using the NPS and customized NPS. Since DANPOS was a necessary algorithmic module in the differential analysis, it is interesting to run the whole analysis pipeline using DANPOS alone without any a priori nucleosome detection steps. The differential analysis of nucleosome positioning (see examples in Supplementary Figs 10a, 11a and 12a ) between the resting and activated CD4+ T cells, reveals that the NPS algorithm only detects a few enriched pathways (fails in this task; Supplementary Fig. 10b ). Yet all the other three algorithms (iNPS, customized NPS and DANPOS) basically detect the same set of enriched pathways, among which iNPS’ enrichment level is the highest ( Fig. 6b , Supplementary Figs 11b and 12b ). Likewise, in terms of predicting enriched motifs, the enrichment level by iNPS ( Fig. 6b ) is again significantly higher than NPS ( Supplementary Fig. 10b ) and customized NPS ( Supplementary Fig. 11b ), but is slightly lower yet at the same level of DANPOS ( Supplementary Fig. 12b ). For the transcription factor network analysis, the size of the largest component for the iNPS-derived network ( Fig. 6c,d , empirical P -value 10 −4 ) is much larger than that from NPS ( Supplementary Fig. 10c,d , empirical P -value=0.0942) and customized NPS ( Supplementary Fig. 11c,d , empirical P -value 10 −4 ), yet comparable with DANPOS ( Supplementary Fig. 12c,d , empirical P -value 10 −4 ). Finally, in the CoCiter’s gene-term analysis, the iNPS-derived transcription factors yield higher average PubMed document counts and more significant P -values than NPS and customized NPS, while the two indices for iNPS and DANPOS are comparable. Taken together, iNPS has better performance in the differential analysis of nucleosome positioning than NPS and customized NPS. Although DANPOS is specifically designed for this purpose and has been shown to be better than other algorithms, we show iNPS yields comparable results with DANPOS and it is even better for predicting biologically significant pathways. Comparison with other software packages We also compared iNPS to other algorithms for nucleosome detection, including NSeq [21] , NucleoFinder [22] , nucleR [23] , NOrMAL [24] , PING [25] , TemplateFilter [26] and DANPOS [10] , using the resting CD4+ T cell MNase-seq data for chromosome 1 (ref. 1 ) (Methods), and compared them with iNPS ( Supplementary Fig. 13 ). NSeq and NucleoFinder detect nucleosomes by finding the centre positions of nucleosomes. These two packages can accurately identify the centre positions of nucleosome peaks ( Supplementary Fig. 13d,e ) but cannot detect the borders of nucleosomes. In contrast, iNPS ( Supplementary Fig. 13b ) provides the range for each nucleosome where the signal is most enriched. nucleR also detects nucleosome positions by finding the summit of peaks after noise filtering, but it is unable to separate nucleosomes well, resulting in inaccurate border determination (compare Supplementary Fig. 13b,f ). NOrMAL and PING detect nucleosome positions based on probabilistic models whose parameters and quantity are estimated from the MNase-seq data. From the profiles on Chromosome 1, these algorithms apparently cannot match the other algorithms ( Supplementary Fig. 13g,h ). In addition, as PING artificially enforced the final width for all the nucleosomes to be 200 bp in the ‘postPING’ step, it sometimes reports adjacent nucleosomes with overlapping positions ( Supplementary Fig. 13h ). Moreover, NOrMAL could only detect nucleosomes on a small chromosomal fragment. In the tests, we had to divide the total sequencing tags of chromosome 1 into >100 parts at ‘nucleosome deserts’ (long chromosome regions >1,000 bp without MNase-seq coverage) (Methods) and run the programme on every part, which altogether took 6.5 h to finish. TemplateFilter identifies nucleosome locations where the forward and reverse read distributions correlate with a series of model templates. Despite the high accuracy of TemplateFilter ( Supplementary Fig. 13i ), it is only able to detect nucleosomes on a small chromosomal fragment. DANPOS is a pipeline mainly designed for analysing dynamic nucleosome positioning and occupancy. It also contains a crude peak-calling algorithm inside which it cannot determine the borders of nucleosomes precisely. It can well detect sharp peaks, but it is unable to exclude noise between peaks ( Supplementary Fig. 13j ). As more quantitative measurements, we compared the distribution of nucleosome widths ( Supplementary Fig. 13k ) and the distribution of distances between two neighbouring nucleosome centres ( Supplementary Fig. 13l ) for the nucleosome positioning results on chromosome 1 in resting CD4+ T cells. While iNPS generated a nucleosome width distribution between 70 and 90 bp (peaking at 80 bp; Supplementary Fig. 13k ) and a neighbouring nucleosome centre distance between 160 and 210 bp (peaking at 180 bp; Supplementary Fig. 13l ), the other algorithms generated more diffuse and flattened distributions with ambiguous maximum (except the distribution of the neighbouring nucleosome centre distances generated by DANPOS). To compare the quality of nucleosome output by different algorithms, we first performed Poisson tests for all the detected nucleosomes. Then, we compared the average −log10( P -value) of nucleosomes (per 10,000-sized bins) for the top 500,000 predicted nucleosomes (on Chromosome 1 of the resting CD4+ T cells) by each algorithm. It is clear that iNPS outperformed all other algorithms against which it was compared ( Fig. 7a,b ). Paired t -tests between iNPS and other algorithms show a significantly higher −log10( P -value) for iNPS detection than other algorithms ( Supplementary Table 5 ). Compared with the differences among different algorithms, there are relatively very small differences among the stepwise results of iNPS, and all these steps yield better nucleosome detection quality than the other algorithms. 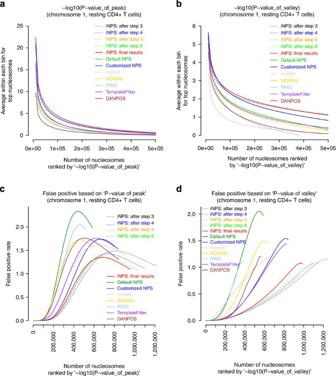Figure 7: Comparison of the nucleosome detection quality and false positive rates among different steps of iNPS and other algorithms on chromosome 1 of the resting CD4+ T cells. Solid lines: iNPS and other algorithms; Dotted lines: the stepwise results of iNPS. (a,b) Significance of the tag distribution in peak or valley of detected nucleosomes. (a) Peak regions, quantified by ‘−log10(P-value_of_peak)’ and (b) valley regions, quantified by ‘−log10(P-value_of_valley)’. The top 500,000 nucleosomes output by each algorithm are used and the average −log(P-value) per 10,000 nucleosomes are plotted. (c,d) Comparison of false positive rate based on ‘P-value of peak’ (c) and ‘P-value of valley’ (d), evaluated by comparing the number of nucleosomes detected from real and randomly simulated MNase-seq data sets. Thexaxis is the number of top ranked nucleosomes predicted by each algorithm, and theyaxis is the false positive rates. Each point on a curve is the average false positive based on 10 times of simulation, and the s.d. is not plotted since they are very small (about 10−4–10−3). Significance of the differences of nucleosome detection quality (a,b)/false positive rates (c,d) between different algorithms is quantified by pairedt-tests, shown inSupplementary Tables 5 and 6, respectively. Figure 7: Comparison of the nucleosome detection quality and false positive rates among different steps of iNPS and other algorithms on chromosome 1 of the resting CD4+ T cells. Solid lines: iNPS and other algorithms; Dotted lines: the stepwise results of iNPS. ( a , b ) Significance of the tag distribution in peak or valley of detected nucleosomes. ( a ) Peak regions, quantified by ‘−log10( P -value_of_peak)’ and ( b ) valley regions, quantified by ‘−log10( P -value_of_valley)’. The top 500,000 nucleosomes output by each algorithm are used and the average −log( P -value) per 10,000 nucleosomes are plotted. ( c , d ) Comparison of false positive rate based on ‘ P -value of peak’ ( c ) and ‘ P -value of valley’ ( d ), evaluated by comparing the number of nucleosomes detected from real and randomly simulated MNase-seq data sets. The x axis is the number of top ranked nucleosomes predicted by each algorithm, and the y axis is the false positive rates. Each point on a curve is the average false positive based on 10 times of simulation, and the s.d. is not plotted since they are very small (about 10 −4 –10 −3 ). Significance of the differences of nucleosome detection quality ( a , b )/false positive rates ( c , d ) between different algorithms is quantified by paired t -tests, shown in Supplementary Tables 5 and 6 , respectively. Full size image Furthermore, it is also important to show this improvement is not accompanied by an increase in the false positive rates by iNPS. Since it is hard to know the ground truth of nucleosome positioning in the genome, to quantify the likelihood of different algorithms to yield false positive nucleosome predictions, we generated synthetic MNase-seq data sets by performing randomized simulations (see Supplementary Table 3 / Supplementary Fig. 3e (dotted purple line) for the numbers/sharpness of nucleosome peaks detected by iNPS on the simulated data) and used the ratio of the number of detected nucleosomes in the synthetic data versus real data as a surrogate measure of ‘false positive rates’ (Methods). From the surrogate ‘false positive rate’ curves (based on ‘ P -value of peak’ or ‘ P -value of valley’; Fig. 7c,d ), it is clear that the iNPS algorithm has the lowest ‘false positive rates’ among all the algorithms compared. Paired t -tests between iNPS and other algorithms show a significantly lower false positive rate for iNPS detection than other algorithms ( Supplementary Table 6 ). This firmly demonstrates that iNPS enjoys the lowest false positive rates in calling nucleosome peaks. Moreover, the false positive rates for the intermediate steps of iNPS are also consistently lower than other algorithms. Specifically, when comparing the performance of these steps, we found that at high x axis values (representing nucleosomes with lower significance), Step 7’s false positive rates are lower than Step 3 when considering peaks yet slightly higher when considering valleys. This observation is consistent with the operation that we filter out some low-quality peaks in Step 4–Step 7 so that the peaks’ quality is improved at the cost of the valleys’. Moreover, a further detailed comparison of iNPS with the other packages ( Table 1 ) indicates an overall advantage of iNPS, which includes well-detected nucleosomes, unambiguous nucleosome positions with ‘steep slopes’ as clear borders, sharp distributions of neighbouring distances, detailed feature descriptions for each detected nucleosome (for example, height, area under the curve and isolated/merged peaks determination) and user convenience. Table 1 Comparison of iNPS with other nucleosome-positioning algorithms. Full size table Four types of nucleosomes identified by iNPS According to the shapes of detected nucleosome peaks, iNPS is able to identify four main types of nucleosomes—‘MainPeak’ (an isolated ‘main’ nucleosome peak), ‘MainPeak+Shoulder’ (a ‘main’ peak associated with a ‘shoulder’), ‘MainPeak:doublet’ (a merged ‘doublet’) and ‘Shoulder’ (an independent ‘shoulder’). Each type of nucleosome has a distinctive distribution of nucleosome width (length between two inflection points of each detected nucleosome peak; Supplementary Fig. 14a,b ), and each kind of neighbouring nucleosome pair (four nucleosome types have altogether 10 kinds of neighbouring nucleosome pair) has a distinct distribution of neighbouring centre distance ( Supplementary Fig. 14c,d ). Compared with the ‘MainPeak’ nucleosomes, which account for ~80% of the detected nucleosomes, the ‘Shoulder’ nucleosomes have a shorter width and closer distance to nearby nucleosomes, while the ‘MainPeak+Shoulder’ and ‘MainPeak:doublet’ nucleosomes are wider between inflection boundaries and farther from nearby nucleosomes ( Supplementary Fig. 14c,d ). These observations suggest that these non-‘MainPeak’ nucleosomes are perhaps associated with nucleosome destabilization. As the histone variant H2A.Z [27] , [28] , [29] or transcription factor binding [30] , [31] , [32] , [33] often induces nucleosome shift or destabilization, we examined the average H2A.Z profiles and average transcription factor motif density profiles around every nucleosome (−1,000 to +1,000 bp) for each type of nucleosome (Methods; Fig. 8 ). Unlike the other two types, the average profiles for the doublet types (‘MainPeak+Shoulder’ and ‘MainPeak:doublet’) have an H2A.Z/nucleosome peak at the centre position (see the green and red lines in Fig. 8a ), indicating enrichment of H2A.Z at these two types of non-‘MainPeak’ nucleosomes. Moreover, the transcription factor motif density distribution has a unique phase for the doublet nucleosomes: for each of the two types of nucleosomes, the highest transcription factor motif density peaks overlap with the nucleosomes (green and red lines in Fig. 8b ), while for ‘MainPeak’ nucleosomes, or other well-phased nucleosomes on either side of any nucleosome, the average transcription factor motif density profile has two high peaks at the valley flanking the nucleosome ( Fig. 8b ). This suggests that doublets are more likely to be associated with ‘on-site’ transcription factor binding on the nucleosome, consistent with their role as mobile or destabilized nucleosomes. We further separately examined the average H2A.Z profiles and average transcription factor motif density profiles for nucleosomes of different distances to the nearest TSS (≤2, 2–10, 10–100 and >100 kb; Supplementary Figs 15 and 16 ). These profiles are consistent with the patterns observed based on the total nucleosome profiles. Taken together, the nucleosome types identified by iNPS based on detected nucleosome shapes also implicate different biological functions of nucleosomes. 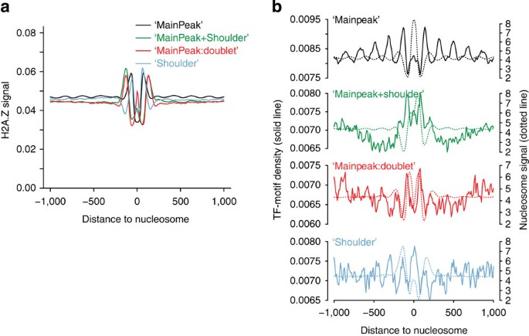Figure 8: Average H2A.Z and transcription factor motif density profiles for the four types of nucleosomes identified by iNPS. (a) Average H2A.Z profiles. (b) Average transcription factor (TF) motif density profiles (solid lines). Nucleosome profiles are also shown as dotted lines for TF-motif enrichments comparison inb. Figure 8: Average H2A.Z and transcription factor motif density profiles for the four types of nucleosomes identified by iNPS. ( a ) Average H2A.Z profiles. ( b ) Average transcription factor (TF) motif density profiles (solid lines). Nucleosome profiles are also shown as dotted lines for TF-motif enrichments comparison in b . Full size image Deep genome sequencing after MNase digestion (MNase-seq) has been an effective way for inferring a genome-wide map of nucleosome positions, in which deriving nucleosome profiles from sequence tags is a key step. In iNPS, we followed NPS to represent the core part of a nucleosome using the middle 75 bp in each 150 bp-extended tag, since taking either full length or the middle point would probably result in a decrease of nucleosome resolution ( Supplementary Fig. 13a ) or a decrease of signal enrichment level. To facilitate further peak calling, a step of profile smoothening could reduce noise. There are various kinds of tactics available, such as Fast Fourier Transform methods used in nucleR [23] and the wavelet- and convolution-based method used in NPS [4] . In practice, we found that the Gaussian convolution method alone was sufficiently effective for profile smoothing. In addition, combining Gaussian convolution with basic derivative operations (convolution with first, second (Laplacian) and third derivatives of Gaussian) in iNPS could correspondingly detect max/min-extremum points (summit/valley), inflection points and the most winding positions on the smoothed profiles. These key locations play important roles in nucleosome positioning: the inflection points identify borders of nucleosomes, the max/min-extremum points help to distinguish the ‘main’ nucleosome candidates and the most winding positions play a part in fate-decision for the ‘shoulder’ candidates. After finishing the basic step of nucleosome detection, iNPS adjusts nucleosome borders of the preliminary results, merges closely located ‘doublets’ and filters some small peaks with bad shapes. With these additional procedures, the final results show increased accuracy ( Fig. 3a,b ) together with a sharper distribution of nucleosome width and neighbouring distances ( Fig. 3e,f ). Different from other packages, iNPS uses both statistical scores (‘−log10( P -value_of_peak)’ and ‘−log10( P -value_of_valley)’) and geometrical features (peak height, peak width and area under the curve) of the detected nucleosome peaks to quantify the confidence level of each nucleosome, which not only increases the detection consistency but also provides further biological insights such as the distinction between well-fixed nucleosomes and potentially destabilized nucleosomes. On the basis of the whole genome-wide nucleosome positioning by iNPS in both resting and activated CD4+ T cells, we found that the differentially positioned nucleosomes are highly enriched for immune pathways ( Fig. 6b ) and for transcription factors, which coherently interact with each other ( Fig. 6c ), which are otherwise not possible to identify using NPS ( Supplementary Fig. 10b,c ). This highlights the great importance of precisely detecting the nucleosome positions. We also compared the consistency and boundary resolution of nucleosome detection between iNPS and NPS. In terms of consistency, our iNPS algorithm could detect the nucleosome-positioning profiles between two independent subsets of MNase-seq data with a SCC 0.489±0.029 (average±s.d. for the 24 chromosome in resting CD4+ T cells), which increased significantly from NPS’s 0.339±0.039 ( P =3.37 × 10 −21 ; Fig. 5a ). In terms of boundary resolution, the nucleosome detected by iNPS has a much sharper width distribution than NPS, with a twofold peak height of that by NPS, and an average width±s.d. of 84.312±15.056 bp and 83.960±15.150 bp (around the peak-region of 40–130 bp for resting and activated T cells, respectively) by iNPS versus 89.913±17.778 bp and 88.864±17.614 bp by NPS, indicating significantly reduced variation of the iNPS detection results (F-test P -value=0; Fig. 3e ). Thus, a better nucleosome detection algorithm, such as iNPS, will definitely enhance the application of MNase-seq technology in various fields of biological research. Finally, a good software tool should be convenient for users. A primary requirement is the direct applicability of the software on a large chromosome and preferably a whole genome. In this respect, iNPS successfully performed nucleosome positioning on the whole human genome but NOrMAL and TemplateFilter could not. Furthermore, the installation and execution of iNPS is easy on the Linux system. Taken together, the improved iNPS algorithm, compared with the original NPS, showed a significantly higher sensitivity, detection quality, robustness and lower false positive rate in detecting genome-wide nucleosome positions from the MNase-seq data. Further comparison of iNPS with other software packages indicated an overall advantage of iNPS, including higher accuracy with clear nucleosome borders, higher detection coverage with better quality, lower false positive rates, more uniform neighbouring distance, more detailed result descriptions for downstream analysis and better user convenience. Data sets and software package Tag coordinate bed files for MNase-digest sequencing data of human CD4+ T cells [1] was downloaded from National Heart Lung and Blood Institute (NHLBI), National Institutes of Health (NIH) ( http://dir.nhlbi.nih.gov/papers/lmi/epigenomes/hgtcellnucleosomes.aspx ). Tag coordinate bed file for H2A.Z ChIP-seq data of human CD4+ T cells [34] was downloaded from NHLBI, NIH ( http://dir.nhlbi.nih.gov/papers/lmi/epigenomes/hgtcell.aspx ). Gene expression microarray data for human CD4+ T cells [1] was downloaded from the GEO repository with accession number GSE10437. Coordinate information of TSSs was downloaded from the UCSC repository ( http://hgdownload.cse.ucsc.edu/goldenPath/hg18/database/refFlat.txt.gz ) on 30 July 2012. The coordinate information of CTCF-binding sites [35] was downloaded from http://bioinformatics-renlab.ucsd.edu/rentrac/wiki/CTCF_Project , and converted into hg18 system. Human protein network data was downloaded from STRING (version 9.05) ( ftp://string-db.org/STRING/9.05/protein.links.detailed.v9.05.human_only.txt.gz ) on 5 August 2013. A predicted transcription factor motif coordinates map for lymphoblastoid cell lines [36] was downloaded from the ‘CENTIPEDE’ website ( http://centipede.uchicago.edu/data/CentipedeAllP99.bed.gz ). For software packages, NPS (Nucleosome Positioning from Sequencing), version 1.3.2, was downloaded from http://liulab.dfci.harvard.edu/NPS/ on 1 December 2011. NSeq [21] was downloaded from https://github.com/songlab/NSeq on 19 April 2013. NucleoFinder [22] was downloaded from https://sites.google.com/site/beckerjeremie/ on 22 April 2013. nucleR [23] , version 1.9.0, was downloaded from http://bioconductor.org/packages/devel/bioc/html/nucleR.html on 25 April 2013. NOrMAL [24] version beta2, was downloaded from http://code.google.com/p/normal-nucleosome-mapping-algorithm/downloads/list on 22 April 2013. PING [25] , Version 2.3.1, was downloaded from http://www.bioconductor.org/packages/devel/bioc/html/PING.html on 28 April 2013. TemplateFilter [26] was downloaded from http://compbio.cs.huji.ac.il/NucPosition/TemplateFiltering/Home.html on 22 April 2013. DANPOS [10] , version 2.1.2, was downloaded from http://code.google.com/p/danpos/ on 14 May 2013. Algorithmic steps in iNPS iNPS is developed based on Zhang et al .’s methods [4] , from which we adopted two key steps—‘nucleosome scoring’ (generating continuous wave-form signal for genome-wide nucleosome positioning) and ‘Laplacian of Gaussian (LoG) convolution’ (detecting inflection points to find candidate nucleosomes). We then designed and integrated our new steps to develop the iNPS algorithm ( Fig. 2b ), including the following eight steps. Step 1—nucleosome scoring . Wave-form nucleosome signal profile, with a resolution of 10 bp, is obtained by extending each sequencing tag (each tag is extended from its 5′ end by 150 bp (~1 nucleosome length) toward its 3′ direction ( Fig. 2b inset)), of which the middle 75 nt was taken to represent the enrichment of nucleosome signal. The nucleosome score at each coordinate is summed by all the extended tags covering this coordinate, and these tags on either sense or antisense strand contribute equally to the score at this coordinate. Step 2—Gaussian convolution . Discrete Gaussian convolution is performed as equation (1) to smoothen the wave-form nucleosome signal profile: where x is the coordinate on the genome, f ( x ) is the original nucleosome scoring at coordinate x , y ( x ) is the smoothed signal at coordinate x , deviation σ =3 and the range ( x –3σ, x +3σ) is used for profile smoothening. σ =1 is also used to generate another mildly smoothed profile for the ‘borders adjustment’ in Step 5. Besides this basic step, convolutions with Gaussian derivatives are also performed to detect important sites on the wave-form profile: 1. Convolution with the first derivative of Gaussian is used as equation (2) to detect max/min-extremum points of the smoothed profile (where the convolution results=0, σ =3): 2. Convolution with the second derivative (Laplacian) of Gaussian (LoG) is used as equation (3) to detect inflection points of the smoothed profile (where the convolution results=0, σ =3), representing the candidate position of nucleosome peaks (See the formula below). This operation is also repeated for ( σ =1) to detect another set of inflection points on the mildly smoothed profile for border adjustment in Step 5. 3. Convolution with the third derivative of Gaussian is used as equation (4) to detect the ‘most winding positions’ of the smoothed profile (where the convolution results=0, σ =3), especially for the ‘shoulder’ patterns: Step 3—candidates identification . A pair of inflection points is identified as a ‘main’ nucleosome candidate if it has a max-extremum point located between them, otherwise it would be identified as a ‘shoulder’ candidate. Step 4—determining shoulder nucleosomes . Every shoulder candidate is determined as an independent nucleosome or the dynamic shifting part of the neighbouring ‘main’ nucleosome candidate, based on the relationship between itself and its neighbour, which includes the distance, peak height ratio between them and profile shape features between the nearest inflection point on the adjacent ‘main’ nucleosome peak and the ‘most-winding’ point (detected by the third derivative of Gaussian convolution) on the ‘shoulder’ ( Fig. 2a ). The profile shape features include the concavity/convexity level of the Gaussian smoothed profile (high concavity level suggests that a shoulder is likely to be an independent nucleosome) and the correlation between original and smoothed profile (high correlation level is indicative that a shoulder is more likely to be a dynamic part of the adjacent nucleosome; see examples in Supplementary Fig. 2 ). Step 5—inflection border adjustment . Some relatively ‘big’ nucleosome peaks would probably affect the border detection (using inflection points) of their neighbouring nucleosomes with ‘small’ peaks. Thus, inflection points on the mildly smoothed profile (LoG with σ =1 in Step 2) are used to adjust the borders of these ‘small’ nucleosome peaks. Step 6—merging doublet nucleosomes . Each ‘doublet’, a pair of extremely closely distributed adjacent peaks with similar height, is merged as one nucleosome. It is based on the relationship between the two neighbouring peaks, which includes the neighbouring centre-to-centre distance, length of the ‘valley’ region (the genomic region between the right inflection point of the left peak and the left inflection point of the right peak), peak height ratio between them and the convex level of the Gaussian smoothed profile in the ‘valley’ region. These criteria are implemented in Step 6 ( Supplementary Table 7 ). If any criterion is satisfied, a pair of adjacent peaks is merged to form a ‘doublet’ ( Supplementary Fig. 17 , see Supplementary Note 1 for details, and see examples in Supplementary Fig. 18 ). Step 7—filtering . Some small nucleosome peaks with bad shapes are discarded. This step is based on the level of concavity (the average LoG) of the peak, the length between two inflection points, and the length of the longest segment with a negative LoG within a peak and so on. We implement six alternative criteria in this step ( Supplementary Table 8 ). If any criterion is satisfied, a detected peak is judged to be of low quality and filtered out subsequently ( Supplementary Fig. 17 , see Supplementary Note 2 for details, and see examples in Supplementary Fig. 19 ). Step 8—statistical evaluation . For each detected nucleosome, the chromosome region between two inflection points is defined as the peak, while the two flanking chromosome regions between one inflection point of this nucleosome and the nearest flanking inflection point of its neighbouring nucleosome are defined as the valley (To avoid unbound valley in the nucleosome desert regions, the maximal size of a valley is set to 1,000 bp). We use the upper- and lower-tailed Poisson test to estimate the enrichment and the depletion levels of sequence tags in the peak and valley regions, respectively. Each MNase-seq tag is extended to 150 bp long from the 5′ to the 3′ direction. The centre of the 150 bp region is used to represent the genomic coordinate of the tag in the Poisson test. Specifically, we compute the number of sequence tags whose genomic coordinates fall into a nucleosome peak or into a valley region. We use Poisson test to estimate the probability of more than (or equal to) the number of observed tags located in a peak region (resulting in a P -value of peak), or less than (or equal to) the number of observed tags located in a valley region (resulting in two P -values for the left/right flanking valleys, respectively). To be conservative in calculating the P -values for a peak region, the maximum tag density of the symmetrically extended 1, 5 or 10 kb genomic regions is computed and then scaled by the length of the peak region as the background tag counts. Conversely, the minimum tag density of the extended 1, 5 or 10 kb genomic regions is used for the test of a valley region. For convenience, we define ‘−log10( P -value_of_peak)’ of a nucleosome as the significance level of a nucleosome peak; ‘−log( P -value_of_valley)’ of a nucleosome as the significance level of the two flanking valleys of a peak, where ‘ P -value of valley’ is simply the geometric mean of the P -values of the two flanking valley regions. Evaluating false positive rate The first step to quantify false positive rates of nucleosome detection is to estimate the confidence level of the peak and flanking valley regions of each detected nucleosome. This is achieved by performing upper and lower-tailed Poisson tests to assess the tag enrichment and depletion in the two regions, resulting in ‘ P -value of peak’ and ‘ P -value of valley’, respectively. Then, given a fixed P -value cutoff, surrogate ‘false positive rates’ of nucleosome detections can be quantified by the ratio of the expected number of ‘false positive’ detections from simulated data versus the number of ‘true’ detections from the actual MNase-seq data. For this purpose, we use chromosome 1 of the resting CD4+ T cell to simulate 10 matched synthetic MNase-seq data sets. This is achieved by dividing the chromosome into 100,000-bp windows and randomly shuffling tag positions in each window. Then, by setting cutoffs with decreasing ‘−log10( P -value)’ scores for nucleosomes detected from the real data, we generate two false positive rate curves, each focusing on the significance of peak and valley regions, respectively. To avoid inaccurate estimation, the rate is only calculated when the denominator is larger than 500, and the P -value cutoffs are upper-bounded by 0.99 to exclude degenerated nucleosomes with no flanking valley (typically outputted by PING, DANPOS and nucleR) from the analysis. Robustness evaluation of nucleosome detection algorithms The input MNase-digest sequencing data set was randomly and evenly divided into two subsets, each containing 50% tags. Then, the same nucleosome-positioning algorithm was run on the two subsets separately, generating two sets of corresponding ‘subresults’. After that, the robustness of the algorithm was quantified for the similarity between the two subresults, by SCC, as follows: First, we computed the ‘nucleosome detection profile’ for each subresult by keeping the wave-form signal within the detected nucleosome peaks and excluding other parts of signal profiles (as the red line in Figs 1b and 3b ). Then, we calculated the SCC value between two nucleosome detection profiles (for example, the orange and the green line in Fig. 3c,d ) to quantify the similarity of the two subresults. Nucleosome detection around TSSs or CTCF-binding sites The gene expression microarray data (GSE10437) for human resting CD4+ T cells [1] was used to select genes with high, medium and low transcription levels, respectively. For any gene (represented by one or a set of RefSeq IDs) with more than one microarray probe, the median value of these probes at each sample was taken as the transcription level for this gene. In total, 18,295 genes with explicit TSS coordinate information in the UCSC repository were collected and ranked by transcription level. Then, three sets of genes with 5% highest, 5% medium and 5% lowest transcription level were selected. For each set of genes, the average ‘nucleosome detection profile’ (with s.d.) around TSSs (−2,000 to +2,000 bp) were plotted with 10 bp resolution. For CTCF-binding sites, we first mapped the genomic coordinates of the CTCF-binding sites in ref. 35 to hg18. Then, the average ‘nucleosome detection profile’ (with s.d.) around all 31,683 sites (−1,000 to +1,000 bp) were plotted at 10 bp resolution. Note that different from TSSs, the regions of CTCF-binding sites do not have ‘upstream’ or ‘downstream’, so every CTCF-binding region was mapped from lower to higher genome coordinates. Testing other software packages For NPS, the parameters for the ‘peak finding’ steps were reset to lower the thresholds or to switch off the filtering ( Supplementary Table 1 ), while the other parameters were set by default. NSeq was tested with default setting except the parameter ‘−f’ is set to 1 (no FDR cutoff) and ‘−t’ is set to 20 (run with 20 cores). NucleoFinder needs a reads count file and a control file as input, so we used an almost empty document as control file here, and all the other settings were kept default. nucleR was tested following its instructions on commands, according to which the key parameters were set as the following: in the ‘processReads’ step, ‘type’ was set to ‘single’ (single-end sequencing), ‘fragmentLen’=147 and ‘trim’=73; in the ‘filterFFT’ step (denoising step), ‘pcKeepComp’ was set to 0.01; in the ‘peakDetection’ step, ‘threshold’ was set to 25% as recommended and ‘width’ was set to 147; in the ‘mergeCalls’ step, ‘min.overlap’ was 50, ‘discard.low’ was 0.2 and ‘mc.cores’ was 1, respectively, as recommended. To test NOrMAL, we divided the total sequencing tags of chromosome 1 at ‘nucleosome deserts’ (long chromosome regions >1,000 bp without MNase-seq coverage) into 115 parts, each part containing ~5 × 10 4 forward/reverse tags, and then, performed nucleosome detection step-by-step. PING was tested by following the provided R code sample in the user’s guide: all the parameters were set according to recommendation, except that ‘nCores’ was set to 20 (run with 20 cores) in the ‘PING-analysis’ step. TemplateFilter was also tested step-by-step (as NOrMAL), with parameters ‘-corr_bound’=0.5 (correlation score bound), ‘-min_width’=80 (minimum nucleosome width), ‘-max_width’=180 (maximum nucleosome width) and ‘-overlap’=0 (no overlap between adjacent nucleosomes). DANPOS was tested with parameters ‘-q,--height’=1 (the intensity cutoff for nucleosome calling), ‘-z,--smooth_width’=100 (the smooth width before peak calling), ‘-e,--edge’=1 (detect edges for peaks), ‘-k,--keep’=1 (save middle stage files), ‘-x,--pcfer’=1 (do nucleosome calling), ‘-n,--nor’=N (no normalization), ‘--frsz’=150 (setting the average size of DNA fragment to 150 bp) and ‘--clonalcut’=0 (don’t adjust clonal signal). Identifying and analysing differential nucleosomes Genome-wide nucleosome positions of resting or activated CD4+ T cells were obtained by running iNPS on the respective MNase-seq datasets [1] . Then, the MNase-seq tags within each extended nucleosome peak region (extending 50 bp on either side) were selected and inputted into DANPOS [10] to obtain differentially positioned nucleosomes. DANPOS was run with parameters ‘-q,--height’=1 (the intensity cutoff for nucleosome calling), ‘-z,--smooth_width’=100 (the smooth width before peak calling), ‘-e,--edge’=1 (detect edges for peaks), ‘-k,--keep’=1 (saving mid-stage files), ‘-x,--pcfer’=0 (no nucleosome calling), ‘-n,--nor’=N (no normalization), ‘--frsz’=150 (setting the average size of DNA fragment to 150 bp) and ‘--clonalcut’=0 (don’t adjust clonal signal). At each peak location of the signal, DANPOS provided a set of P -values and false positive rates (FDRs) to score the difference of nucleosome signal between resting and activated CD4+ T cells. The locations meeting any one of the following two criteria, (1) ‘point_diff_FDR’≤0.01 with a determined ‘diff_smt_loca’ or (2) ‘smt_diff_FDR’≤0.05, were determined as the significantly different nucleosomes between resting and activated CD4+ T cells (see the example fragment in Fig. 6a ). Then, a 2,000-bp sliding window was moved across the genome with a 500 bp step size to select the windows enriched with differentially positioned nucleosomes (~ top 1% windows that have ≥5 differentially positioned nucleosomes were selected). The differentially positioned nucleosomes in the windows were used for GREAT (Genomic Regions Enrichment of Annotations Tool) (Version 2.02) analysis [37] to calculate statistical associations of these nucleosomes with nearby (proximal −10 to +10 Kbp) genes (including TSS and curated regulatory domains) and to provide enriched biological functional terms (FDR<0.05 and region-based fold ≥2). To examine the functional coherence of the transcription factors whose motifs are most enriched (hypergeometric test FDR<0.001 by GREAT) in the iNPS-detected differentially positioned nucleosomes, we used the functional interaction network among these transcription factors (constructed by STRING online tool, Version 9.05, http://string-db.org/ ). Then, the biological significance of the transcription factor network was evaluated by using CoCiter’s [38] (Version 1.1, http://www.picb.ac.cn/hanlab/cociter ) ‘gene-term’ analysis for all the transcription factors in the network against two terms ‘T-cell activation’ and ‘activated T cell’. H2A.Z and transcription factor motif density profiles For each 10 bp bin within –1,000 to +1,000 bp around each nucleosome, the raw H2A.Z signal is normalized by the nucleosome signal using the following formula: For transcription factor motif density, genome-wide coordinates of transcription factor motifs [36] were mapped to the −1,000 to +1,000 bp windows around each nucleosome with a 10 bp resolution. How to cite this article: Chen, W. et al . Improved nucleosome-positioning algorithm iNPS for accurate nucleosome positioning from sequencing data. Nat. Commun. 5:4909 doi: 10.1038/ncomms5909 (2014).